Correspondence: Spontaneous secondary mutations confound analysis of the essential two-component system WalKR inStaphylococcus aureus Bacteria and molecular tools The S. aureus UoM Newman was obtained from Professor Tim Foster (Trinity College Dublin); NRS384 was obtained from BEI resources ( www.beiresources.org ). S. aureus was routinely grown in Tryptic Soy Broth (TSB-Oxoid) at 37 °C with aeration at 200 r.p.m. 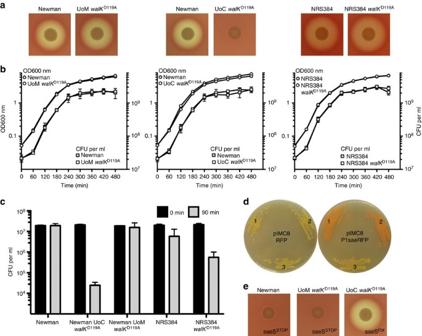Figure 1: Phenotypic screening ofwalKEC-PASmutants. (a) No impact on haemolysis was observed for the WalKD119Amutation in either Newman or NRS384 on sheep blood agar. (b) Growth kinetics were identical for the newly created WalKD119Amutants in TSB at 37 °C with aeration (200 r.p.m.) when compared with the parental strain. Optical density (○) and colony-forming units (□) were enumerated. (c) In a lysostaphin growth sensitivity assay, the UoC WalKD119Aexhibited a loss of viability, while the parent or UoM WalKD119Adid not. The WalKD119Amutation in the NRS384 background enhanced sensitivity to lysostaphin when compared with the parental strain. Error bars depict the s.d. of the mean from three independent experiments. (d) P1 sae promoter activity with a DsRED reporter. Left: no promoter. Right: P1 sae driving RFP expression; (1) Newman (2) UoM WalKD119A(3) UoC WalKD119A. No expression ofsaewas observed in UoC WalKD119A. (e) By allelic exchange, the UoCsaeSmutation was introduced into Newman or UoM WalKD119A(saeSSTOP) with haemolysis abolished, while introduction of the wild-typesaeSgene into UoC WalKD119A(saeSFIX) restored haemolysis. Primers were purchased from IDT ( www.idtdna.com ) with primer sequences detailed in Supplementary Table 1 . Restriction enzymes, Phusion DNA polymerase and T4 DNA ligase were purchased from New England Biolabs. Genomic DNA was isolated from 1 ml of an overnight culture (DNeasy Blood and Tissue Kit—Qiagen) pretreated with 100 μg of lysostaphin (Sigma cat. no. L7386). DHBP was purchased from Sigma (cat. no. 126217; 100 g). Lysostaphin sensitivity assay Overnight cultures of S. aureus were diluted 1:100 in fresh, prewarmed TSB in the presence of 0.2 μg ml −1 of lysostaphin with or without 75 μM DHBP (100 mM stock in methanol). Broths were incubated statically at 37 °C. Colony-forming units were determined by spot plate dilution on Brain heart infusion agar (Difco) at 0 and 90 min. Limit of detection for the assay was 10 3 CFU ml −1 . Construction of pIMC8-RFP and SLiCE cloning The S. aureus codon optimized DsRED red fluorescent protein and upstream TIR sequence from pRFP-F (ref. 12 ) was PCR amplified with primers IM314/IM315. The product was digested with KpnI/SacI and cloned into the complementary digested pIMC8 (non-temperature-sensitive version of pIMC5 (ref. 13 )), creating pIMC8-RFP. To clone into pIMAY-Z [3] and pIMC8-RFP, primers were tailed with 30 nt of complementary sequence to the plasmid. Amplimers were inserted with seamless ligation cloning extract (SLiCE; ref. 14 ) into the vector (pIMAY-Z: walRK D119A , sae STOP , sae FIX ; pIMC8-RFP: P1 sae). Either vector was linearized with KpnI, gel extracted and PCR amplified with primers IM1/IM2 (pIMAY-Z) or IM1/IM385 (pIMC8-RFP). Both amplimers (vector and insert) were combined in a 10 μl reaction containing 1 × T4 ligase buffer, with 1 μl of SLiCE extract. The reaction was incubated at 37 °C for 1 h and then transformed into Escherichia coli strain IM08B [3] , with selection on Luria agar plates containing chloramphenicol 10 μg ml −1 . Plasmids were extracted and directly transformed by electroporation into the target S. aureus strain [3] . Production of SLiCE extract The SLiCE was isolated from DY380 (ref. 14 ) grown in 50 ml 2xYT (1.6% Tryptone, 1% Yeast Extract, 0.5% NaCl) at 30 °C after a 1:100 dilution of the overnight culture. Once the culture reached an OD 600 of ∼ 2.5, the cells were moved to 42 °C for 25 min (addition of 50 ml of 42 °C 2xYT). Cells were processed as described by Zhang et al . [14] , with the pellet lysed in 500 μl of CelLytic B cell lysis reagent (C87040; 10 ml; Sigma). Whole-genome sequencing and data analysis Whole-genome sequencing was performed using the Illumina NextSeq (2 × 150 bp chemistry), with library preparation using Nextera XT (Illumina). Resulting reads were mapped to the S. aureus Newman reference (Accession: NC_009641) using Snippy v3.1 ( https://github.com/tseemann/snippy ). Note that 89 substitutions, 20 deletions and 25 insertions were shared between UoC and UoM Newman strains compared with the NC_009641 reference sequence, representing likely sequencing errors in the 2008 published reference [2] . Data availability All sequencing data used in this study have been deposited in the National Center for Biotechnology Information BioProject database and are accessible through the BioProject accession number PRJEB14381 ( https://www.ncbi.nlm.nih.gov/bioproject/325902 ). An updated S. aureus Newman genome sequence is available (Genbank reference: NZ_LT598688.1). How to cite this article: Monk, I. R. et al . Correspondence: Spontaneous secondary mutations confound analysis of the essential two component system WalKR in Staphylococcus aureus . Nat. Commun . 8, 14403 doi: 10.1038/ncomms14403 (2017). Publisher’s note : Springer Nature remains neutral with regard to jurisdictional claims in published maps and institutional affiliations.